Isolation and characterization of a covalent CeIV-Aryl complex with an anomalous13C chemical shift The synthesis of bona fide organometallic Ce IV complexes is a formidable challenge given the typically oxidizing properties of the Ce IV cation and reducing tendencies of carbanions. Herein, we report a pair of compounds comprising a Ce IV − C aryl bond [Li(THF) 4 ][Ce IV (κ 2 - ortho -oxa)(MBP) 2 ] ( 3-THF ) and [Li(DME) 3 ][Ce IV (κ 2 - ortho -oxa)(MBP) 2 ] ( 3-DME ), ortho -oxa = dihydro-dimethyl-2-[4-(trifluoromethyl)phenyl]-oxazolide, MBP 2– = 2,2′-methylenebis(6- tert -butyl-4-methylphenolate), which exhibit Ce IV − C aryl bond lengths of 2.571(7) – 2.5806(19) Å and strongly-deshielded, Ce IV − C ipso 13 C{ 1 H} NMR resonances at 255.6 ppm. Computational analyses reveal the Ce contribution to the Ce IV − C aryl bond of 3-THF is ~12%, indicating appreciable metal-ligand covalency. Computations also reproduce the characteristic 13 C{ 1 H} resonance, and show a strong influence from spin-orbit coupling (SOC) effects on the chemical shift. The results demonstrate that SOC-driven deshielding is present for Ce IV − C ipso 13 C{ 1 H} resonances and not just for diamagnetic actinide compounds. The bonding between lanthanides and ligands has been described as purely ionic [1] , [2] . However, modern spectroscopic and computational techniques have challenged this simple assumption [3] , [4] , [5] , [6] . The covalency in M − X interactions can result in anomalous and diagnostic nuclear magnetic resonance shifts, X = 13 C, 15 N, 19 F, 77 Se, 125 Te, resulting from participation of f-element orbital angular momentum [7] , [8] , [9] , [10] , [11] , [12] , [13] . Another important aspect of detailed f-element electronic structure is multiconfigurational character, as described in the model example of cerocene, Ce(COT) 2 , COT = cyclooctatetraene ligand [14] . The case for multiconfigurational character in cerocene has been made through X-ray absorption, SQUID magnetometry, and multi-reference computational studies and tied strongly to the characteristics of the cerium-carbon bonding [15] . Despite the interest surrounding f-element covalency and multiconfigurational effects, there are few examples of organometallic Ce IV complexes [16] . The current literature is limited to metallocene Ce IV complexes or α-heteroatom stabilized Ce IV − C σ-bonds. Reported examples of Ce IV − metallocene bonding include Ce IV complexes of cyclopentadienide, cyclooctatetraene dianion, and bispentalene dianion ligands [17] , [18] , [19] , [20] , [21] . Complexes containing a Ce IV − C σ-bond, however, are limited to either an N -heterocyclic carbene (NHC) complexes, e.g., Ce[L 4 ] (Fig. 1a ), or a bis(iminophosphorano)methandiide complex, e.g., [Ce(BIPM TMS )(ODipp) 2 ] (Fig. 1a ) [22] , [23] . The latter examples are expected to have electronic structures that deviate significantly from typical organometallic alkyl, aryl, or alkynyl ligands due to the heteroatom α-substitution [22] , [23] , [24] , [25] . The scarcity of Ce IV − C containing-complexes likely arises from the unstable combination of strongly reducing carbanions and the oxidizing Ce IV cation [16] . As a result, the formation of reactive, carbon-centered radicals and Ce III species is observed. Our team has a long-standing interest in the isolation of redox stable Ce IV species to elucidate the relationship between ligand field and the Ce III /Ce IV couple [26] , [27] , [28] . Fig. 1: Examples of Ce IV − C σ bonds. a Previous examples of complexes with formally Ce IV − C σ bonds, which are stabilized by either nitrogen [22] or phosphorus heteroatoms [23] . b This work detailing the synthesis and characterization of a Ce IV − C aryl bond, including computational analysis. Carbon atoms bound to cerium are indicated with a C . Full size image Herein, we expand our studies for the isolation of a pair of Ce IV − C aryl compounds. These compounds display unusually high 13 C NMR shifts compared to other diamagnetic M IV − C aryl compounds. Relativistic density functional calculations verify that the high NMR shifts are due to large SOC effects supported by the increased covalency of the Ce IV − C aryl bond. Synthesis and structures of Ce IV − C aryl Considering strategies to stabilize a Ce IV − C aryl bond, we hypothesized that tethering the aryl group to the Ce center would kinetically inhibit homolysis of the Ce − C bond. In addition, we sought a sterically-protected Ce center to prevent reactivity at the ipso -carbon. Lastly, we chose a supporting ligand that would stabilize the Ce IV oxidation state to prevent charge transfer and subsequent Ce − C bond homolysis. With these considerations in mind, we aimed to prepare a Ce IV − C aryl bond from the Ce IV bis(methylene bisphenolate) complex Ce(THF) 2 (MBP) 2 , that was previously synthesized by members of the Schelter laboratory ( 1 , Fig. 2 ) [29] . Aryloxide ligands have been previously shown to both stabilize the Ce IV oxidation state and high valent organometallic species of other metal species [28] , [29] , [30] , [31] , [32] , [33] , [34] . Addition of a yellow solution of ortho -lithiated oxazoline 2 (Li- ortho -oxa) to a purple benzene solution of Ce(THF) 2 (MBP) 2 ( 1 ) at room temperature resulted in an immediate color change of the solution to dark red. The 1 H NMR spectrum of the reaction mixture revealed loss of the pseudo C 2v symmetry of 1 and formation of a C 1 symmetric product. Likewise, there was also a shift in both the 7 Li and 19 F NMR resonances of 2 , and the two methylene protons and methyl groups of the oxazoline were no longer degenerate in the 1 H NMR spectrum. All 1 H, 7 Li, and 19 F NMR resonances were well within the range of diamagnetic signals, leading to the assignment of the product of the reaction as [Li(THF) 4 ][Ce(κ 2 - ortho -oxa)(MBP) 2 ] ( 3-THF ). Dark red X-ray quality crystals of 3-THF were grown over 3 days from a cooled (−25 °C) mixture of 3-THF in toluene and THF layered with pentane. The crystals were collected in 66% yield (Fig. 2 ). Alternatively, crystallizing from a cooled (−25 °C) solution of crude 3-THF in DME layered with pentane resulted in dark-red X-ray quality crystals of 3-DME over 3 days (Fig. 3 ). Crystals of 3-DME were collected in a slightly higher 75% yield. The differences in NMR data between 3-THF and 3-DME are negligible compared to experimental error. While compound 3-DME crystallizes with a single molecule in the asymmetric unit, compound 3-THF crystallizes with two independent molecules in the asymmetric unit, with only minor differences between the structures. The Ce − O(phenoxide) bond distances of 3-THF and 3-DME (2.1636(13)–2.202(4) Å) compare well with the Ce − O(phenoxide) bond distances observed in the reported structure of 1 (2.113(2)–2.152(2) Å) [29] . The Ce − C bond distances of 3-THF and 3-DME are 2.571(7) – 2.5806(19) Å and are shorter than reported Ce III − C aryl bond lengths: 2.621(4) – 2.64 ± 0.02 Å [35] , [36] . The difference in ionic radii between 6-coordinate Ce III and Ce IV is 0.14 Å; however, the difference between 3-THF and 3-DME and previous Ce III − C aryl complexes is only 0.04 – 0.07 Å [37] . We ascribe this difference to the steric demand by the MTB ligands vs. the pentamethylcyclopentadienyl ligands used in the prior work. Previously reported complexes containing Ce IV − C σ-bonds are 2.652(7) – 2.705(2) Å and 2.385(2) – 2.441(5) Å for the Ce − C NHC and Ce − C(bis(iminophosphorano)methandiide) ligands, respectively [22] , [23] , [25] . With this data in hand, we assign this complex as a Ce IV − C aryl complex. Fig. 2: Syntheses of title Ce IV − C aryl compounds 3-THF and 3-DME. The complex 1 was treated with the isolable aryl lithium 2 to generate the title complexes 3-THF or 3-DME . Full size image Fig. 3: Crystal structure of 3-DME. Thermal ellipsoid plot of the X-ray crystal structure of 3-DME at the 30% probability level. For clarity, C–H hydrogens and the Li(DME) 3 + cation were removed; In addition tert -butyl groups are displayed in wireframe. Selected bond lengths in Å: Ce(1)–C(9): 2.5806(19); Ce(1)–N(1): 2.6176(16); Ce(1)–O(2): 2.1750(12); Ce(1)–O(3): 2.2062(13); Ce(1)–O(4): 2.1640(12); Ce(1)–O(5): 2.1636(13). Full size image Electrochemical analysis To better understand how the ortho -oxa − group impacts the stability of the Ce IV cation, electrochemistry was performed on 3-THF . The E pa of 3-THF , −1.67 V vs. Fc/Fc + , shifts by −0.72 V relative to the E 1/2 of 1 (−0.94 V vs. Fc/Fc + ), indicating that the ortho -oxa − moiety significantly stabilizes the Ce IV couple in THF. The reduction of 3-THF is not reversible under the electrochemical conditions, although the event precedes a reversible oxidation at E 1/2 = −0.94 V vs. Fc/Fc + and an irreversible oxidation at E pa = −0.43 V (Supplementary Figs. 18 – 19 ). We postulate that the reduction of the Ce IV center is followed by dissociation of the ortho -oxa − fragment, producing 1 and 2 . Indeed, the return anodic scan comprises waves at E 1/2 = −0.94 V vs. Fc/Fc + and E pa = −0.43 V respectively, consistent with the previous assignment for compound 1 and inferred for compound 2 (Fig. 4 ) [29] . Fig. 4: Cyclic voltammagram of 3-THF. Solvent: THF; electrolyte 0.1 M [ n Pr 4 N][BAr F 4 ]; [analyte] = 0.001 M; OCP = −0.815 V vs. Fc/Fc + , noted by the right-facing arrow; ν = 100 mV s −1 . The trace shows the reduction of 3 at E pc = −1.67 V vs. Fc/Fc + with a return wave at E 1/2 = −0.94 V vs. Fc/Fc + , which is the Ce III /Ce IV couple of 1 [29] . The waves corresponding to 1 do not appear in the first scan (Supplementary Figs. 18 – 19 ). Full size image 13 C NMR analysis While the 1 H, 7 Li, and 19 F NMR of 3-THF and 3-DME showed minimal changes compared to the starting materials, the 13 C{ 1 H} NMR of the ipso -carbon of both 3-THF and 3-DME showed a significant shift (difference between 3-THF and 3-DME is less than >0.05 ppm which is within error). Indeed, the ipso - 13 C{ 1 H} resonance was located at 255.6 ppm, well outside of the typical range for aryl resonances (100–170 ppm) and shifted by ~50 ppm downfield relative to the Li − C aryl resonance for the starting material, 2 (Fig. 5 ). This 13 C{ 1 H} shift is further downfield than observed for other characterized, diamagnetic M IV − C aryl interactions; the highest being Th(2-C 6 H 4 CH 2 NMe 2 ) 4 , which exhibits a Th IV − C 13 C{ 1 H} signal at 230.8 ppm [38] , [39] . The shift of the 13 C{ 1 H} signal for the carbon atom bound to metal cations has been implicated as a reporter for the degree of covalency in f-element cation-carbon bonds [7] , [8] , [9] . In this light, 3-THF and 3-DME have an anomalously high covalency for a M IV -aryl interaction. As with the bond distance metrics, there are few salient examples of Ce IV − C σ-bonds for comparison of the 13 C{ 1 H} NMR shifts. The compounds isolated by P. Arnold and co-workers display a 13 C{ 1 H} shift at ~213 ppm for the Ce IV –NHC [22] . The compounds reported by Liddle contain Ce IV − C (bis(iminophosphorano)methandiide) 13 C{ 1 H} shifts in the range of 324.6–343.5 ppm, depending on the secondary ligands bound to the Ce IV cation; [Ce(BIPM TMS )(ODipp) 2 ] exhibits a 13 C{ 1 H} shift of 324.6 ppm [23] , [25] . Notably, these compounds contain substantially different substituents attached to the Ce– C carbon, diminishing the significance of their comparison. Fig. 5: Identification of the unusual 13 C resonance. A portion of the HMBC spectrum showing the long-range C-H coupling to the 13 C resonance at 255.6 ppm. An interpretation of the spectrum is inlaid, indicating that the signal at 255.6 ppm corresponds to the ipso -carbon. Full size image Computational bonding analysis To further understand the nature of the Ce IV − C aryl interaction, we turned to computations to assess the electronic structure of the anionic, cerium-containing portion of 3-THF (referred to as 3 ). The geometry of 3 was optimized starting from the structure of 3-THF determined by X-ray crystallography, using density functional theory (DFT) with the B3LYP functional, all-electron Slater-type basis sets for all atoms, and other standard settings as detailed in the SI. The agreement between experiment and theory was excellent, with only minor differences in the Ce IV − ligand bond lengths (≤0.02 Å). The MOs with the most Ce 4f character remain largely metal-centered and span the seven lowest unoccupied molecular orbitals (LUMO to LUMO + 6, Supplementary Figs. 13 – 19 ) of the complex, a common feature for Ce IV compounds as well as for cerium species with a debated Ce IV /Ce III oxidation state [3] , [15] . HOMO to HOMO − 3 (Supplementary Figs. 26 – 29 ), for 3 are mostly delocalized phenoxide-centered orbitals, while HOMO − 4 (Fig. 6 ) corresponds to the highest occupied orbital showing significant ligand-metal (Ce IV − C aryl ) hybridization. Fig. 6: MO’s of 3 depicting the Ce–C aryl bond. a The DFT/B3LYP frontier Kohn-Sham molecular orbital of 3 (HOMO − 4). b The two-center two-electron bonding NLMO. 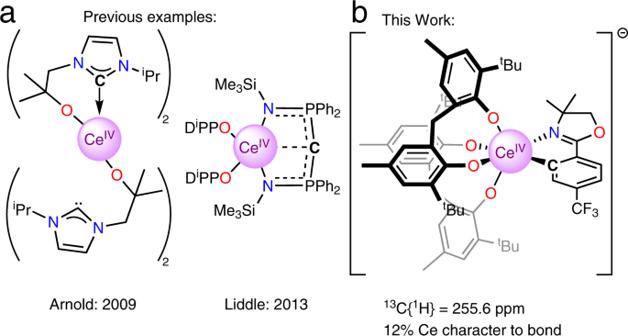Fig. 1: Examples of CeIV− C σ bonds. aPrevious examples of complexes with formally CeIV− C σ bonds, which are stabilized by either nitrogen22or phosphorus heteroatoms23.bThis work detailing the synthesis and characterization of a CeIV− Carylbond, including computational analysis. Carbon atoms bound to cerium are indicated with aC. Atomic orbital contributions of the NLMOs and other bond properties of all the Ce containing bonds are listed in Table 1 . Full size image The metal-ligand bonding in 3 is characterized in Fig. 6 and Table 1 in terms of natural localized molecular orbitals (NLMOs) and bond orders. There are two two-center two-electron σ bonds describing the donation bonding between the aryl carbon and oxazolinide nitrogen and Ce, and σ + 2π bonds describing the bonding between each of the O atoms and Ce (Supplementary Figs. 37 – 40 ). Among these, the Ce IV − C aryl σ bond shown in Fig. 6 has the largest covalency, in terms of shared density, with 12% Ce contribution of which 32/62% involve 5d/4f. Previously reported Ce IV − C bonds contain 8–13% Ce contribution [25] . Ce tends to be less covalent than U VI (U VI − C bonds 22–29% U) but similar to Th IV (Th IV − C aryl bonds 10–15%) [9] , [25] , [38] , [40] . In the remaining σ and π bonds with the N and O atoms, Ce contributes about 3–4% weight, suggesting that these bonds are mainly ionic. The bond ionicities are also reflected in the bond orders compiled in Table 1 , all being significantly smaller than one (which would indicate a full single bond). In the sum of all interactions, however, Ce receives sizable electron donation from the surrounding ligands. For instance, the calculated Ce charge is +2.26 (Mulliken charge), +2.46 (Bader charge), and +2.44 (natural charge from a natural bond orbital (NBO) analysis) instead of the formal +4. The Ce natural electron configuration retrieved from the NBO analysis is 4f 0.76 d 0.60 , which deviates considerably from the formal 4f 0 5d 0 . The large Ce 4f electron count of 3 (0.76), associated mainly with the sizable Ce − C aryl bonding, is comparable to the calculated and experimentally-determined Ce 4f electron counts in CeO 2 and Ce(C 8 H 8 ) 2 [41] , [42] , [43] . We anticipate that this similarity has important implications regarding the electronic structure of 3 , in the sense that it may potentially exhibit a multi-configurational ground-state wavefunction with Ce III/IV character, similar to cerocene. However, further spectroscopic studies are needed, and are under way, to confirm this assignment for 3 . Table 1 NLMO compositions and bond orders for 3. 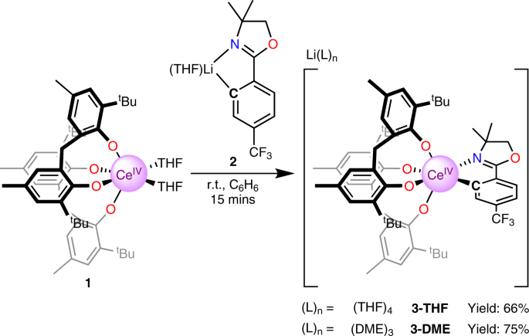Fig. 2: Syntheses of title CeIV− Carylcompounds 3-THF and 3-DME. The complex1was treated with the isolable aryl lithium2to generate the title complexes3-THFor3-DME. Full size table Computational chemical shift analysis Computed 13 C NMR chemical shifts for the ipso -carbon, with various approaches, are compiled in Supplementary Table 2 . The NMR shift was sensitive to the applied DFT approximations, a common observation in NMR shift calculations for compounds containing lanthanides and actinides. The best agreement with the experiment (256 ppm) for the ipso - 13 C chemical shift in 3 was obtained with a PBE hybrid with 40% exact exchange, PBEh-40, which gave 259 ppm. The same functional previously provided excellent ligand chemical shifts in actinide complexes [40] , [44] . PBEh-40 produced a similar cerium electronic structure (Mulliken/natural charge of +2.43/+2.66, 4f 0.58 5d 0.59 NBO natural electron configuration, Ce − C aryl WBO of 0.37) as B3LYP. Reasonable agreement with the experimental chemical shift was obtained also with the KT2 functional (265 ppm), which is known to perform well in NMR calculations [45] . The comparison between the ipso - 13 C chemical shift calculated without and with SOC, with PBEh-40/KT2, reveals a 40/51 ppm downfield shift caused by SOC, which is largely triggered by the Ce 4f and 5d involvement in the Ce IV − C aryl σ bond. In order to rationalize the anomalous 13 C shift, we carried out an analysis of the DFT/PBEh-40 13 C isotropic shielding (σ iso ) in terms of NLMOs [46] , [47] . The NMR shielding data are gathered in Table 2 and the relevant NLMOs are shown in Supplementary Fig. 41 . Note that these NLMOs are equivalent to those obtained with DFT/B3LYP. The analysis shows that the σ(Ce − C aryl ) covalent bond is the principal cause of the SOC-induced deshielding of the ipso -carbon. According to Table 2 , the core orbital of the Ce-bound C aryl brings a diamagnetic contribution of roughly 200 ppm to σ iso . This value is counterbalanced by two large, negative shielding contributions generated by the σ bonds involving the ipso -carbon, namely the σ(Ce − C aryl ) bond and the two σ(C aryl − C) bonds involving the two neighboring carbons of the aryl ring, denoted as C 1 and C 2 . From Table 2 it is evident that the σ(Ce − C aryl ) contribution to σ iso is as important (without SOC) or even more important (with SOC) than the combined σ iso contributions generated by the σ(C aryl − C) NLMOs. Table 2 NLMO contributions to the 13 C isotropic nuclear shielding (σ iso ) in 3 a . Full size table Indeed, with SOC in particular, the σ(Ce − C aryl ) NLMO yields a dominant negative contribution to σ iso of −154 ppm, of which −169 ppm is paramagnetic and 15 ppm is diamagnetic (not shown separately in Table 2 ), while the combined σ iso contribution from the σ(C aryl − C 1,2 ) NLMOs is −99 ppm. The overall SOC effects on the total isotropic shielding, σ iso , add up to −39 ppm. The largest contribution to this value is generated by the σ(Ce − C aryl ) NLMO, −52 ppm, and there are secondary contributions from the σ(C aryl − C 1,2 ) NLMOs, 11 ppm (Table 2 , last column), indicating that these orbitals are somewhat delocalized onto the metal. Hence, the covalent bonding between the Ce center and C aryl is the main contributor of the 13 C SOC deshielding and this aspect is strongly related to the sizable Ce 4f and 5d character of the σ(Ce − C aryl ) NLMO: 53% f and 41% d with PBEh-40, or 62% f and 32% d with B3LYP, with the 4f likely generating most of the SOC deshielding. We have synthesized, characterized, and crystallized complexes featuring a Ce IV − C aryl bond. The synthesis of the title complexes 3-THF and 3-DME was realized from the reaction of the lithium-aryl salt 2 with 1 . Electrochemical analysis revealed that the aryl interaction resulted in a notable stabilization of the Ce IV oxidation state, shifting the E pc of Ce IV reduction by 720 mV relative to the THF adduct. A combination of 13 C{ 1 H} NMR and DFT was used to investigate the covalency of the Ce IV − C aryl bonding. 13 C{ 1 H} NMR analysis revealed that the ipso -carbon was shifted to 255.6 ppm, an indicator of metal-ligand covalency in the Ce IV − C aryl bond. This result was supported by NLMO analysis, which showed a 12% metal contribution to the Ce IV − C aryl bond. We expect that these results will further inform fundamental bonding in high valent f-elements and be effective in guiding the preparation of other f-element organometallic complexes. General considerations See Supplementary Methods for further details. Ce(THF) 2 (MBP) 2 (1) We previously reported a synthesis of 1 that could not be separated from the lithium halide byproducts [29] . This revised method provides clean 1 . In an N 2 filled drybox, to a clear, colorless solution of H 2 MBP (0.270 g, 0.793 mmol, 2 equiv) in 4 mL of THF in a 20 mL scintillation vial with a Teflon coated stir bar, was added a yellow solution of Ce(O t Bu) 4 (THF) 2 (0.200 g, 0.396 mmol, 1 equiv) in a 6 mL solution of 2:1 THF:benzene at room temperature with stirring. The reaction immediately turned an intense purple color and was stirred for 1 h. The volatile materials were removed under reduced pressure, the residue was triturated with 2 mL of benzene to liberate the tert -butanol byproduct, and the volatile materials were again removed under reduced pressure. The resulting purple solid was transferred onto a medium porosity fritted filter and washed with 5 × 2 mL of pentane. The purple solid was dried under reduced pressure for 3 h. Yield: 0.311 g, 0.324 mmol, 82%. NMR data for this complex was not previously reported and is provided here: 1 H NMR (400 MHz, THF- d 8 ) δ: 7.15 (s, 4H), 6.79 (s, 4H), 5.01 (d, J = 13.4 Hz, 2H) 3.51 (d, J = 14.0 Hz, 2H), 2.31 (s, 12 H), 1.44 (s, 36 H). 13 C{ 1 H} NMR (100 MHz, THF- d 8 ) δ: 168.12, 137.25, 134.45, 129.13, 128.17, 124.12, 35.40, 34.99, 31.15, 20.93. The quantity of THF present for 1 was verified by 1 H-NMR in C 6 D 6 . [Li(THF)][ ortho -oxa] (2) Synthesis adapted from similar compounds [48] . In a N 2 filled drybox, a solution containing H- ortho -oxa (1.217 g, 5.0 mmol, 1 equiv) and 10 mL of hexanes in a 20 mL scintillation vial with a Teflon coated stir bar was placed in a −30 °C freezer for 30 mins. The vial was removed from the freezer and, while stirring, a solution of n- butyl lithium (2.5 M, 5 mmol, 2 mL) was added dropwise over 5 min. The solution turned from colorless to yellow to brown and a yellow solid precipitated. The reaction mixture was stirred for 50 min at room temperature, after which the solid was collected by filtration over a coarse-porosity fritted-filter and subsequently washed with 3 × 2 mL of hexanes and 1 × 2 mL of pentane. The tan solid was then dried under reduced pressure for 2 h. The solid was then dissolved in minimal THF at rt and then placed in a −30 °C freezer overnight. Yellow crystalline blocks formed and were collected over a coarse-porosity fritted-filter and washed with 3 × 2 mL of pentane. The yellow blocks were dried for 2 h under reduced pressure. Yield: 0.831 g, 2.59 mmol, 52%. 1 H NMR (400 MHz, THF- d 8 ) δ: 8.28 (s, 1H), 7.57 (d, J = 8.0 Hz, 1H), 7.07 (dd, J = 8.0, 2.7 Hz, 1H), 4.17 (s, 2H), 1.34 (s, 6H). 13 C{ 1 H} NMR (101 MHz, THF- d 8 ) δ: 203.98, 172.88, 143.18 (q, J = 2.2 Hz), 137.45 (q, J = 3.3 Hz), 127.47 (q, J = 274.1 Hz), 127.31 (q, J = 28.2 Hz), 124.46, 119.28 (q, J = 4.0 Hz), 80.39, 66.58, 29.03. 19 F NMR (376 MHz, THF- d 8 ) δ: –64.29 7 Li NMR (156 MHz, THF- d 8 ) δ: 2.08 Anal. Cal. for C 12 H 11 F 3 LiNO•(C 4 H 8 O) 0.5 : C, 58.96; H, 5.30; N, 4.91. Found C, 59.41; H, 5.41; N, 4.75. The quantity of THF present for 2 was verified by 1 H-NMR in C 6 D 6 . [Li(THF) 4 ][Ce(ortho-oxa)(MBP) 2 (3-THF) In an N 2 filled drybox, two 20 mL scintillation vials were placed in a −30 °C freezer. One contained a dark purple solution of 1 (0.200 g, 0.208 mmol, 1 equiv) in 4 mL of benzene with a Teflon coated stir bar and the other contained a yellow solution of 2 (0.067 g, 0.208 mmol, 1 equiv) in 4 mL of benzene. After cooling for 30 min, the now frozen solution of 2 was removed from the freezer and allowed to thaw. Immediately upon thawing, the frozen solution of 1 was removed from the freezer and the solution of 2 was added dropwise at rt over 2 min. Upon mixing, the solution immediately changed from a dark purple to a dark red color and was allowed to stir for 5 min at rt. At this point the volatile materials were removed under vacuum. The resulting solid was redissolved in a mixture of 3 mL of toluene and 8 drops of THF in an 8 mL scintillation vial. This solution was layered with 5 mL of pentane and placed in a −30 °C freezer for 3 days. During this time, red crystals formed, and were collected by filtration over a medium porosity fritted filter and washed with cold pentane 5 × 2 mL. Yield: 0.198 g, 0.137 mmol, 66%. 1 H NMR (500 MHz, THF- d 8 ) δ: 8.53 (s, 1H), 7.78 (d, J = 8.0 Hz, 1H), 7.12 (d, J = 7.5 Hz, 1H), 7.01 (s, 2H), 6.92 (s, 2H), 6.75 (s, 1H), 6.66 (s, 1H), 6.62 (s, 1H), 6.58 (s, 1H), 5.10 (d, J = 13.4 Hz, 1H), 4.72 (d, J = 13.5 Hz, 1H), 4.32 (s, 1H), 4.01 (s, 1H), 3.23 (d, J = 13.4 Hz, 1H), 3.10 (d, J = 13.6 Hz, 1H), 2.27 − 2.05 (m, 12H), 1.57 (s, 3H), 1.45 (s, 9H), 1.39 (s, 9H), 1.24 (s, 3H), 1.16 (s, 9H), 1.08 (s, 9H). 13 C{ 1 H} NMR (126 MHz, THF- d 8 ) δ: 255.58, 174.49, 168.21, 167.40, 166.81, 137.97, 137.72, 137.33, 137.11, 136.98, 136.79, 135.03, 134.90, 134.58, 132.58 (q, J = 3.1 Hz), 131.11 (q, J = 29.3 Hz), 128.85, 128.75, 128.61, 127.02, 126.64 (q, J = 177 Hz), 126.08, 124.25, 124.11, 123.95, 123.60, 120.18 (q, J = 4.1 Hz), 82.35, 68.88, 35.89, 35.71, 35.60, 35.03, 32.46, 31.54, 31.09, 30.97, 30.16, 21.31, 21.17. 19 F NMR (470 MHz, THF- d 8 ) δ: −62.44 7 Li NMR (194 MHz, THF- d 8 ) δ: −0.57 X-ray quality crystals were obtained from a vapor diffusion of pentane into concentrated solutions of 3 in a solution consisting of 1:2 THF:tolulene in a −30 °C freezer. Anal. Cal. for C 74 H 99 CeF 3 LiNO 9 •(C 7 H 8 ): C, 65.61; H, 7.66; F, 3.95; N, 1.03. Found C, 65.21; H, 6.65; N, 1.30. Best result of three attempts. UV-Vis: λ = 460 nm (ε = 7533 Lmol −1 cm −1 ), λ = 292 nm (ε = 24,426 Lmol −1 cm −1 ). [ Li(DME) 3 ][Ce(ortho-oxa)(MBP) 2 (3-DME) In an N 2 filled drybox, two 20 mL scintillation vials were placed in a − 30 °C freezer. One contained a dark purple solution of 1 (0.100 g, 0.104 mmol, 1 equiv) in 2 mL of benzene with a Teflon coated stir bar and the other contained a yellow solution of 2 (0.034 g, 0.104 mmol, 1 equiv) in 2 mL of benzene. After cooling for 30 min, the now frozen solution of 2 was removed from the freezer and allowed to thaw. Immediately upon thawing, the frozen solution of 1 was removed from the freezer and the solution of 2 was added dropwise at rt over 2 min. 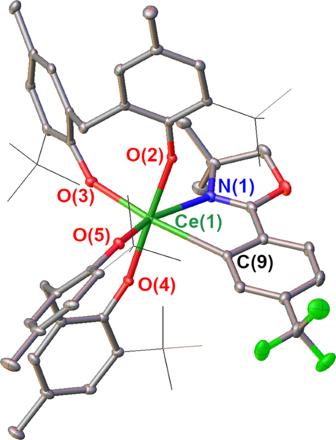Fig. 3: Crystal structure of 3-DME. Thermal ellipsoid plot of the X-ray crystal structure of3-DMEat the 30% probability level. For clarity, C–H hydrogens and the Li(DME)3+cation were removed; In additiontert-butyl groups are displayed in wireframe. Selected bond lengths in Å: Ce(1)–C(9): 2.5806(19); Ce(1)–N(1): 2.6176(16); Ce(1)–O(2): 2.1750(12); Ce(1)–O(3): 2.2062(13); Ce(1)–O(4): 2.1640(12); Ce(1)–O(5): 2.1636(13). Upon mixing, the solution immediately changed from a dark purple to a dark red color and was allowed to stir for 5 min at rt. 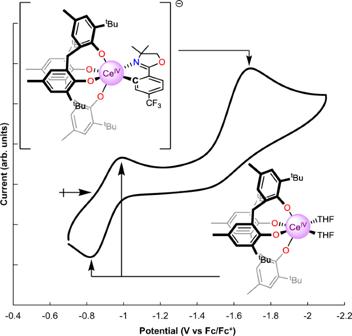Fig. 4: Cyclic voltammagram of 3-THF. Solvent: THF; electrolyte 0.1 M [nPr4N][BArF4]; [analyte] = 0.001 M; OCP = −0.815 V vs. Fc/Fc+, noted by the right-facing arrow; ν = 100 mV s−1. The trace shows the reduction of3atEpc= −1.67 V vs. Fc/Fc+with a return wave atE1/2= −0.94 V vs. Fc/Fc+, which is the CeIII/CeIVcouple of129. The waves corresponding to1do not appear in the first scan (Supplementary Figs.18–19). At this point the volatile materials were removed under reduced pressure. The resulting solid was dissolved in of 3 mL of DME in an 8 mL scintillation vial. This solution was layered with 5 mL of pentane and placed in a −30 °C freezer for 3 days. 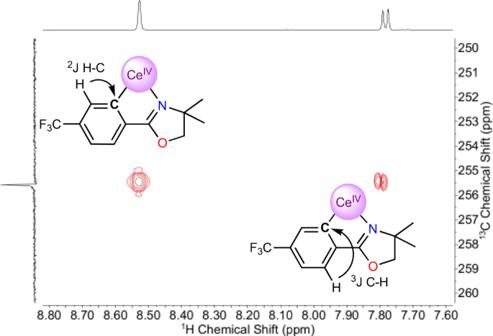Fig. 5: Identification of the unusual13C resonance. A portion of the HMBC spectrum showing the long-range C-H coupling to the13C resonance at 255.6 ppm. An interpretation of the spectrum is inlaid, indicating that the signal at 255.6 ppm corresponds to theipso-carbon. 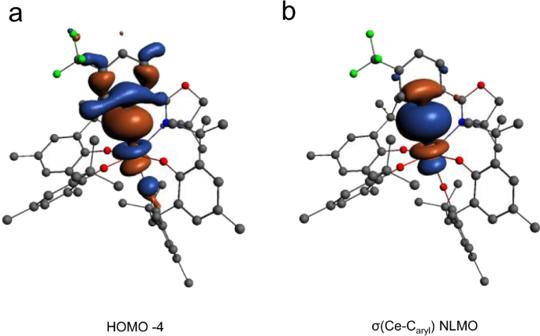Fig. 6: MO’s of 3 depicting the Ce–Carylbond. aThe DFT/B3LYP frontier Kohn-Sham molecular orbital of3(HOMO − 4).bThe two-center two-electron bonding NLMO. Atomic orbital contributions of the NLMOs and other bond properties of all the Ce containing bonds are listed in Table1. During this time, red crystals formed, and were collected by filtration over a medium porosity fritted filter and washed with cold pentane 5 × 2 mL. Yield: 0.111 g, 0.079 mmol, 75%. 1 H NMR (500 MHz, THF- d 8 ) δ: 8.53 (s, 1H), 7.80 (d, J = 7.9 Hz, 1H), 7.13 (dd, J = 8.1 Hz, 2.6 Hz, 1H), 7.01 (s, 2H), 6.91 (s, 2H), 6.76 (s, 1H), 6.68 (s, 1H), 6.64 (s, 1H), 6.59 (s, 1H), 5.12 (d, J = 13.3 Hz, 1H), 4.72 (d, J = 13.4 Hz, 1H), 4.33 (d, J = 7.6 Hz, 1H), 4.01 (d, J = 6.6 Hz 1H), 3.24 (d, J = 13.6 Hz, 1H), 3.11 (d, J = 13.6 Hz, 1H), 2.24 (s, 3H), 2.19 (s, 9H), 1.58 (s, 3H), 1.46 (s, 9H), 1.40 (s, 9H), 1.25 (s, 3H), 1.17 (s, 9H), 1.09 (s, 9H). 13 C{ 1 H} NMR (126 MHz, THF-d 8 ) δ: 255.61, 174.55, 168.23, 167.46, 166.87, 138.03, 137.77, 137.40, 137.18, 137.05, 136.84, 135.08, 134.94, 134.63, 132.65 (q, J = 3.5 Hz), 131.18 (q, J = 29.5 Hz), 129.03, 128.82, 128.66, 127.22 (q, J = 177 Hz), 127.06, 126.14, 124.29, 124.18, 123.99, 123.66, 120.24 (q, J = 4.0 Hz), 82.41, 68.93, 35.94, 35.76, 35.68, 35.09, 32.52, 31.59, 31.14, 31.03, 30.22, 21.36, 21.21. 19 F NMR (470 MHz, THF- d 8 ) δ: −62.44 7 Li NMR (194 MHz, THF- d 8 ) δ: −0.57 X-ray quality crystals were obtained from a layering of pentane on top of a saturated solution of 3-DME in DME (1:1, DME:Pentane). Anal. Cal. for C 70 H 101 CeF 3 LiNO 11 : C, 62.90; H, 7.62; N, 1.05. Found C, 62.45; H, 7.32; N, 1.55.